Structure-guided discovery of potent and dual-acting human parainfluenza virus haemagglutinin–neuraminidase inhibitors Human parainfluenza viruses (hPIVs) cause upper and lower respiratory tract disease in children that results in a significant number of hospitalizations and impacts health systems worldwide. To date, neither antiviral drugs nor vaccines are approved for clinical use against parainfluenza virus, which reinforces the urgent need for new therapeutic discovery strategies. Here we use a multidisciplinary approach to develop potent inhibitors that target a structural feature within the hPIV type 3 haemagglutinin–neuraminidase (hPIV-3 HN). These dual-acting designer inhibitors represent the most potent designer compounds and efficiently block both hPIV cell entry and virion progeny release. We also define the binding mode of these inhibitors in the presence of whole-inactivated hPIV and recombinantly expressed hPIV-3 HN by Saturation Transfer Difference NMR spectroscopy. Collectively, our study provides an antiviral preclinical candidate and a new direction towards the discovery of potential anti-parainfluenza drugs. The Paramyxoviridae family contains viruses that are clinically significant in both medical and veterinary settings [1] . Human parainfluenza viruses types 1 to 3 (hPIV-1, 2 and 3), members of this family, are the leading cause of upper and lower respiratory tract disease in infants and young children and also impact the elderly and immunocompromised [2] , [3] , [4] , [5] . Significantly, it is estimated that in the United States alone, up to five million lower respiratory tract infections occur each year in children who are below 5 years, and hPIV has been isolated in approximately one-third of these cases [6] , [7] . There are currently neither vaccines [8] nor specific antiviral therapy [9] to prevent or treat hPIV infections, respectively, despite continuing efforts [10] . Some of the more recent approaches have focused on an entry blockade [11] and the triggering of premature virus fusion by a small molecule [12] . An initial interaction of parainfluenza virus with the host cell is through its surface glycoprotein, haemagglutinin–neuraminidase (HN) [13] and involves the recognition of N -acetylneuraminic acid ( 1 )-containing glycoconjugates [14] , [15] , [16] ( Fig. 1a ). The parainfluenza virus HN is a multifunctional protein that encompasses the functions of receptor binding (for cell adhesion) and receptor destruction (facilitating virus release), not only within the one protein, but apparently in a single binding site [13] . In addition, the HN is involved in the activation of the viral surface fusion (F) protein necessary to initiate infection of the target host cell [13] , [17] . The essential triple role of HN in viral pathogenesis makes it an ideal target for the development of hPIV-specific therapeutics. A limited number of unsaturated neuraminic acid-based HN inhibitors ( 2 – 6 , Fig. 1a ) have been reported [18] , [19] , [20] , [21] , [22] , [23] , although none of these inhibitors have advanced as clinical candidates presumably due to the lack of sufficient antiviral effect. One of the most potent and widely investigated hPIV type 3 haemagglutinin–neuraminidase (hPIV-3 HN) inhibitors [18] , [20] , [21] to date, 6 , has a neuraminidase IC 50 value of ∼ 20 μM. This inhibitor incorporates an isobutyramido group at C5, demonstrating that hPIV-3 HN can accommodate larger acylamino groups in the C5-binding domain, and an azide functionality at C4 on the unsaturated neuraminic acid-based template. 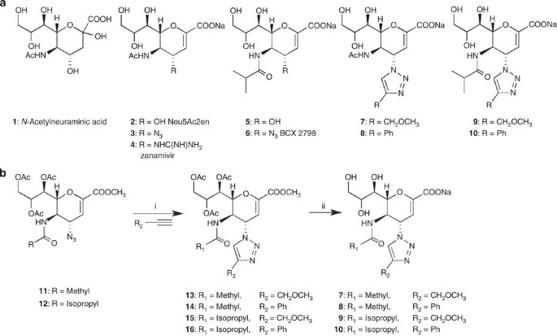Figure 1: Structures of reference sialidase inhibitors, the novel hPIV inhibitors and the synthetic strategy. (a) Structures ofN-acetylneuraminic acid (1), the naturally occurring sialidase inhibitor Neu5Ac2en (2), 4-azido-4-deoxy-Neu5Ac2en (3), the potent influenza virus sialidase inhibitor zanamivir (4), the C5 isobutyramido analogue of Neu5Ac2en (5), the reference hPIV inhibitor BCX 2798 (6) and the novel inhibitors7–10. (b) Synthesis of the novel hPIV inhibitors7–10. (i) CuSO4, sodium ascorbate,tert-butanol/H2O (1:1), 45 °C, 6 h (13, 78%;14, 82%;15, 71%;16, 84%); (ii) NaOH, MeOH/H2O (1:1), RT, o/n (7, 85%;8, 96%;9, 92%;10, 89%). Figure 1: Structures of reference sialidase inhibitors, the novel hPIV inhibitors and the synthetic strategy. ( a ) Structures of N -acetylneuraminic acid ( 1 ), the naturally occurring sialidase inhibitor Neu5Ac2en ( 2 ), 4-azido-4-deoxy-Neu5Ac2en ( 3 ), the potent influenza virus sialidase inhibitor zanamivir ( 4 ), the C5 isobutyramido analogue of Neu5Ac2en ( 5 ), the reference hPIV inhibitor BCX 2798 ( 6 ) and the novel inhibitors 7 – 10 . ( b ) Synthesis of the novel hPIV inhibitors 7 – 10 . (i) CuSO 4 , sodium ascorbate, tert -butanol/H 2 O (1:1), 45 °C, 6 h ( 13 , 78%; 14 , 82%; 15 , 71%; 16 , 84%); (ii) NaOH, MeOH/H 2 O (1:1), RT, o/n ( 7 , 85%; 8 , 96%; 9 , 92%; 10 , 89%). Full size image We have recently described [24] significant flexibility associated with the hPIV-3 HN 216 loop that borders the active site region. This flexible loop can establish a more open cavity, the 216 cavity, and provides new opportunities for inhibitor discovery. Here we successfully explore this exciting opportunity using a multidisciplinary approach that employs, structure-based computational chemistry, synthetic chemistry, NMR-based structural and biological techniques to discover potent inhibitors of hPIV-3 HN activity and cell infection. Computational chemistry and inhibitor design The characterization of the hPIV-3 HN 216 loop flexibility [24] motivated us to explore the potential of designing Neu5Ac2en derivatives with bulky C4 substituents that could be accommodated in and lock open the 216 cavity within the active site. Accordingly, molecular dynamics (MD) simulations have been employed to design and assess Neu5Ac2en derivatives that incorporate C4-functionalized triazoles. From our initial study of 216 loop flexibility and the resultant 216 cavity dimensions, it was clear that relatively bulky C4 substituents on the unsaturated neuraminic acid-based template ( 7 – 10 , Fig. 1a ) could be well tolerated within the open 216 cavity. Furthermore, modelling of these C4 triazole-substituted inhibitors in complex with hPIV-3 HN led us to conclude that both an acetamido ( 7 , 8 ) and an isobutyramido ( 9 , 10 ) moiety at C5 on the template could also be well accommodated simultaneously within the C5-binding domain. We specifically assessed, using MD simulations, the capacity of the bulkier triazole compounds ( 8 and 10 ) to efficiently lock open the 216 loop in hPIV-3 HN. Finally, we determined relative interaction energies of 8 and 10 in complex with hPIV-3 HN to predict if the bulkier C5 acylamino moiety, in combination with the bulky C4 substituent, would be expected to improve inhibitor affinity. Compound 8 as an hPIV-3 HN inhibitor model The simulation of the available hPIV-3 HN crystal structure (PDB accession code 1V3E ) (ref. 25 ) in complex with 8 , using a defined parameter set ( Supplementary Table 1a–e ), allowed an analysis of the dynamic behaviour of the protein relative to the zanamivir ( 4 )-bound structure. Atom-positional root mean square deviations (r.m.s.d.) of the hPIV-3 HN backbone atoms (C α , N, C) for the 216 loop from the simulations of the hPIV-3 HN– 4 and – 8 complexes are presented in Fig. 2a . From this study, it is apparent that the 216 loop undergoes more significant deviations from the crystal structure in the case of the hPIV-3 HN –8 complex (black curve). r.m.s.d. values greater than 0.5 nm are observed for the simulation of the hPIV-3 HN –8 complex, whereas the structure deviates less (0.4 nm) for the hPIV-3 HN –4 complex. 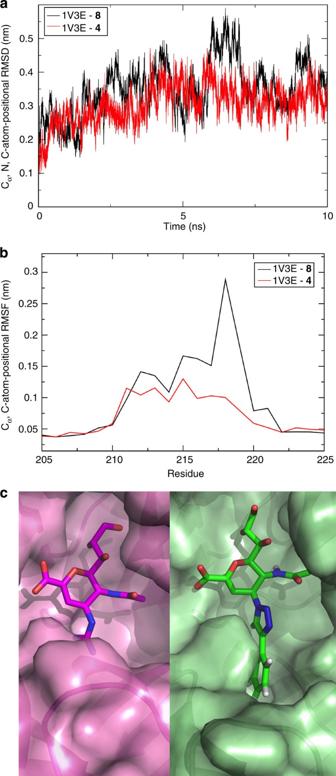Figure 2: The predicted influence of 4 and 8 complexation on HN 216 loop conformation. (a) Atom-positional r.m.s.d. of the 216 loop’s backbone atoms (Cα, N, C) with respect to the crystal structure of hPIV-3 HN (1V3E) bound to zanamivir. (b) Atom-positional r.m.s.f. of the Cαatoms of the residues in the 216 loop, hPIV-3 HN (1V3E) bound to4(red) and hPIV-3 HN (1V3E) bound to8(black). The least-squares superposition involved all Cαatoms of the protein backbone. (c) Solvent-accessible surface plots of the final coordinates of hPIV-3 HN (1V3E) bound to4(left) and bound to8(right).8can be accommodated in an open-loop structure of hPIV-3 HN. Figure 2: The predicted influence of 4 and 8 complexation on HN 216 loop conformation. ( a ) Atom-positional r.m.s.d. of the 216 loop’s backbone atoms (C α , N, C) with respect to the crystal structure of hPIV-3 HN (1V3E) bound to zanamivir. ( b ) Atom-positional r.m.s.f. of the C α atoms of the residues in the 216 loop, hPIV-3 HN (1V3E) bound to 4 (red) and hPIV-3 HN (1V3E) bound to 8 (black). The least-squares superposition involved all C α atoms of the protein backbone. ( c ) Solvent-accessible surface plots of the final coordinates of hPIV-3 HN (1V3E) bound to 4 (left) and bound to 8 (right). 8 can be accommodated in an open-loop structure of hPIV-3 HN. Full size image This notion is further supported by the root mean square fluctuations (r.m.s.f.) observed for the C α atoms of the backbone for residues associated with the 216 loop (residues 205–225, Fig. 2b ). Increased r.m.s.f. are observed for the residues of the second half of the 216 loop (215–220), where values of ∼ 0.3 nm are reached, indicating a substantial conformational rearrangement within that domain compared with the starting hPIV-3 HN reference X-ray crystal structure (PDB accession code IV3E ) (ref. 25 ). Table 1 shows a selection of r.m.s.f. values of residues comprised in the 216 loop. Table 1 Root mean square fluctuations of selected residues comprised in the 216 loop for the 1V3E– 4 and 1V3E– 8 simulated systems, in nanometres, compared with the reference X-ray structure (PDB accession code 1V3E ). Full size table Our data suggest that loop flexibility, present under physiological simulation conditions, has been significantly underestimated in crystal structures and provides an exciting opportunity for anti-parainfluenza virus drug discovery. Comparison of the hPIV-3 HN– 4 complex and the hPIV-3 HN– 8 complex simulations demonstrates that the C4 substituent on 8 induces significant movement in the hPIV-3 HN 216 loop. The induced loop opening can be seen from the solvent-accessible surface plots of the final structures obtained from 10-ns simulations of hPIV-3 HN– 4 complex ( Fig. 2c , left panel) and hPIV-3 HN– 8 complex ( Fig. 2c , right panel). One of the most populated conformational clusters from the MD simulations of hPIV-3 HN in complex with 4 and 8 , are shown in Fig. 3a , while the superposition of the final conformations from the simulations of hPIV-3 HN in complex with 4 and 8 are shown in Fig. 3b . The difference in 216 loop conformation can clearly be seen (coloured loops: 1V3E– 4 (magenta) and 1V3E– 8 (green)). The 216 cavity adopts a more open conformation when in complex with the more sterically encumbered inhibitor 8 . Generally, a wider cavity is observed for the simulation of hPIV-3 HN– 8 complex. The most populated cluster from the simulation of the hPIV-3 HN– 4 complex has a slightly smaller cavity volume (654 Å 3 ) compared with the simulated hPIV-3 HN– 8 complex (717 Å 3 ). 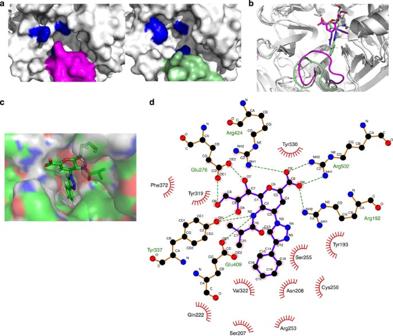Figure 3: The predicted structure of the HN active site in complex with 4 and 8. (a) Solvent-accessible surface plots of the most populated conformational clusters of hPIV-3 HN (1V3E) bound to4(left) and bound to8(right). The residues comprised in the 216 loop (205–225) are coloured in magenta (1V3E–4) and green (1V3E–8), respectively. Arginines associated with inhibitor binding are coloured in blue. (b) Superposition of snapshots of the final trajectories of hPIV-3 HN bound to4and8after 10 ns of MD simulation. The 216 loop is highlighted in colour (green: 1V3E–8, magenta: 1V3E–4).4(magenta) and8(atomic colours) are shown in stick representation. (c) Solvent-accessible surface plot of the final coordinates of hPIV-3 HN (1V3E) bound to10. Both the C4-functionalized triazole and the C5 isobutyramido moiety are well accommodated in an open 216-loop structure of hPIV-3 HN. (d) Key interactions between10and hPIV-3 HN. The triarginyl cluster (Arg192, Arg424, Arg502) engages the inhibitor’s negatively charged carboxylate, the C7 hydroxyl group engages Glu276 in a hydrogen bond interaction as does the C5 isobutyramido NH with Tyr337 and Glu409. Hydrophobic interactions are observed for both the C4 aromatic and C5 isobutyl functionalities. Figure 3: The predicted structure of the HN active site in complex with 4 and 8. ( a ) Solvent-accessible surface plots of the most populated conformational clusters of hPIV-3 HN (1V3E) bound to 4 (left) and bound to 8 (right). The residues comprised in the 216 loop (205–225) are coloured in magenta (1V3E– 4 ) and green (1V3E– 8 ), respectively. Arginines associated with inhibitor binding are coloured in blue. ( b ) Superposition of snapshots of the final trajectories of hPIV-3 HN bound to 4 and 8 after 10 ns of MD simulation. The 216 loop is highlighted in colour (green: 1V3E– 8 , magenta: 1V3E– 4 ). 4 (magenta) and 8 (atomic colours) are shown in stick representation. ( c ) Solvent-accessible surface plot of the final coordinates of hPIV-3 HN (1V3E) bound to 10 . Both the C4-functionalized triazole and the C5 isobutyramido moiety are well accommodated in an open 216-loop structure of hPIV-3 HN. ( d ) Key interactions between 10 and hPIV-3 HN. The triarginyl cluster (Arg192, Arg424, Arg502) engages the inhibitor’s negatively charged carboxylate, the C7 hydroxyl group engages Glu276 in a hydrogen bond interaction as does the C5 isobutyramido NH with Tyr337 and Glu409. Hydrophobic interactions are observed for both the C4 aromatic and C5 isobutyl functionalities. Full size image To evaluate if a bulkier C5 acylamino moiety would be accommodated in the presence of the C4-functionalized triazole, we undertook an identical analysis of 10 in complex with hPIV-3 HN ( Supplementary Movie 1 ). Our preliminary analysis led us to conclude that a C5 isobutyramido moiety is well accommodated within the C5-binding domain in the presence of the C4-functionalized triazole ( Fig. 3c ). Inhibitor-relative interaction energies To quantify the extent of inhibitor engagement with hPIV-3 HN, we have used our MD simulations approach to determine theoretical averaged interaction energies for the known inhibitor 2 , based on a previous study [24] , as well as the novel C5 acetamido and C5 isobutyramido inhibitors, 8 and 10, respectively. Average interaction energy ( E avI ) values of −609.38±10.92, −733.96±15.49 and −821.88±10.93 kJ mol −1 for 2 , 8 and 10 , respectively, in complex with hPIV-3 HN (PDB accession code 1V3E ) (ref. 25 ) were determined. Most importantly, these calculations support the notion that the replacement of the acetamido moiety in 8 with an isobutyramido moiety in 10 significantly improves the absolute E avI value of the inhibitor in complex with the protein. Consequently, 10 is predicted to be a more potent hPIV-3 HN inhibitor than 8 . Further analysis of the MD simulation and extraction of the lowest (−1,078.13 kJ mol −1 ) interaction energy structure of 10 in complex with hPIV-3 HN (1V3E) revealed that 10 makes several key interactions, in this orientation, within the binding pocket ( Fig. 3d ). Noteworthy is the electrostatic interaction between the ligand’s carboxylate and the triarginyl cluster (Arg192, Arg424, Arg502), hydrogen bond interactions between the C7 hydroxyl group and Glu276 and the C5 isobutyramido NH and Tyr337 and Glu409. Furthermore, additional hydrophobic interactions are observed for both the C4 aromatic and C5 isobutyl functionalities, particularly with the peptide backbone, within the C4- and C5-binding domains, respectively. Synthesis of the target triazoles 7–10 Guided by our computational analysis, we synthesized the identified C4-functionalized triazole unsaturated N -acetylneuraminic acid derivatives 7 – 10 to further explore their capacity to inhibit hPIV-3 HN function by accessing an open 216 loop within the hPIV-3 HN-binding site. The synthesis of the triazoles 7 – 10 was achieved using the known [26] , [27] , [28] , [29] 4-azido-4-deoxy-Neu5Ac2en-based intermediates 11 and 12 . Thus, each of the two intermediates was exposed to either methylpropargyl ether or ethynylbenzene under typical click azide–alkyne coupling conditions [27] , [28] (heating a mixture of the 4-azido-4-deoxy-Neu5Ac2en derivative, alkyne, CuSO 4 and sodium ascorbate in a (1:1) mixture of water and tert -butanol for 6 h) to afford the triazole derivative ( Fig. 1b ). Triazoles 13 and 14 (starting from 11 ) and the triazole derivatives 15 and 16 (starting from 12 ) were isolated in yields of 78, 82, 71 and 84%, respectively. The resulting per- O -acetylated triazole derivatives 13 – 16 were then deprotected by treatment with aqueous methanol (50%) adjusted to pH 13–14 at room temperature (RT) for 24 h to yield the final products 7 – 10 as sodium salts in 85, 96, 92 and 89% yields, respectively. The novel compounds were appropriately characterized ( Supplementary Methods ) and all compounds were determined, by 1 H and 13 C NMR spectroscopy, to be of high purity ( Supplementary Fig. 3a–t ). Inhibitor screening with hPIV-3 HN The reference inhibitors 2 , 3 , 5 and 6 , as well as the novel inhibitors 7 – 10 , were evaluated for their capacity to inhibit both the neuraminidase and haemagglutinin functions of the hPIV-3 HN protein using neuraminidase inhibition (NI) and haemagglutination inhibition (HI) assays. Thus, NI was assessed by an end point fluorescence-based assay employing the substrate 2′-(4-methylumbelliferyl) α- D - N -acetylneuraminide (MUN) [18] , [30] , [31] , [32] . The HI evaluation methodology [18] , [33] utilized both guinea pig red blood cells (gp RBC) and human red blood cells (h RBC) to determine virus-mediated agglutination of erythrocytes. A comparison of the potency of the synthesized C4-modified Neu5Ac2en derivatives against hPIV-3 HN was undertaken and, for convenience sake, the IC 50 values were divided into two groups based on the acylamino group present at C5. Group 1 inhibitors have a C5 acetamido functionality and Group 2 inhibitors have a C5 isobutyramido functionality ( Fig. 4 , Supplementary Fig. 4 and Supplementary Table 2 ). The benchmark and well-characterized broad spectrum neuraminidase inhibitor Neu5Ac2en ( 2 ) showed the weakest inhibition with IC 50 values of 1,565 μM and 1,438 μM for hPIV-3 HN NI and HI, respectively. The inhibition observed for 3 , the C5 acetamido analogue of BCX 2798 ( 6 ), was improved when compared with 2 , although it was still in the high micromolar range with IC 50 values of 138 μM and 210 μM for hPIV-3 HN NI and HI, respectively. These IC 50 values were similar to those observed for our novel inhibitor 7 , a C4 methoxymethyl-functionalized triazole Neu5Ac2en derivative, with experimentally determined hPIV-3 HN NI and HI IC 50 values of 154 and 313 μM, respectively. A significant improvement in potency was observed on replacement of the C4 triazole’s methoxymethyl moiety ( 7 ) with a bulkier phenyl group ( 8 ). IC 50 values of 6.5 and 4.6 μM were determined for hPIV-3 HN NI and HI for 8 , respectively. 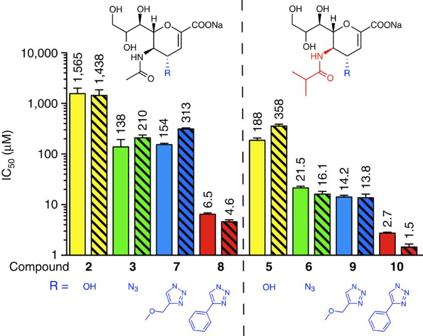Figure 4: NI (solid) and HI (dashed) IC50values for the Neu5Ac2en derivatives2,3,5–10. Inhibitors2,3,7,8with a C5 acetamido group (left panel, group 1) and inhibitors5,6,9,10with a C5 isobutyramido group (right panel, group 2). These values are the means of determinations from three independent experiments and error bars correspond to calculated s.d. Figure 4: NI (solid) and HI (dashed) IC 50 values for the Neu5Ac2en derivatives 2 , 3 , 5 – 10 . Inhibitors 2 , 3 , 7 , 8 with a C5 acetamido group (left panel, group 1) and inhibitors 5 , 6 , 9 , 10 with a C5 isobutyramido group (right panel, group 2). These values are the means of determinations from three independent experiments and error bars correspond to calculated s.d. Full size image In the second group of inhibitors, which contain a C5 isobutyramido functionality, it was obvious that the affinity of each inhibitor was improved relative to its C5 acetamido analogue. The order of potency, not unexpectedly, was identical within the same group. Thus, the weakest inhibition was found for 5 , the C5 isobutyramido analogue of Neu5Ac2en, with IC 50 values of 188 and 358 μM for NI and HI, respectively, and IC 50 values of 21.5 and 16.1 μM for NI and HI, respectively, were determined for the reference hPIV inhibitor BCX 2798 ( 6 ). Inhibitor 9 , with the relatively small methoxymethyl substituent on the triazole ring, had IC 50 values close to those determined for the C4 azido analogue 6 (IC 50 =14.2 and 13.8 μM for NI and HI, respectively). Similarly, as observed in the C5 acetamido-containing Group 1 inhibitors, increasing the substituent size from the methoxymethyl group in inhibitor 9 to a bulkier phenyl moiety as in inhibitor 10 resulted in a remarkable improvement in potency with IC 50 values of 2.7 and 1.5 μM for NI and HI, respectively. Interestingly, an improvement in HI IC 50 values was observed when h RBCs were used instead of gp RBCs ( Supplementary Fig. 5 ). This improvement most likely reflects sialic acid content and/or linkage presentation differences between human and guinea pig red blood cells. For example, it is well known that human tissues and cells, including red blood cells, only express N -acetylneuraminic acid-containing glycoconjugate receptors, whereas other animals also express N -glycolylneuraminic acid-based receptors [34] , [35] . Nevertheless, irrespective of the specific red blood cells used, our designer inhibitor 10 had significantly higher potency when compared with the benchmark compound 6 . Finally, we have also determined ( Supplementary Methods ) a K m value for MUN of 5.1 mM and K i values of 1.3 and 16 μM for inhibitors 10 and 6 , respectively. Cell-based assays Following initial enzymatic screening, the most potent inhibitor 10 and the reference hPIV inhibitor (BCX 2798, 6 ) were then evaluated in a growth inhibition assay to compare their capacity to inhibit hPIV-3 virus infection and propagation in LLC-MK2 cells ( Supplementary Fig. 6 ). Compound 6 was chosen as a reference inhibitor as it is the most documented hPIV-3 Neu5Ac2en-based inhibitor to date and has reasonable in vitro hPIV-3 antiviral potency [18] , [21] . In an initial assay, at an inhibitor concentration of 2 μM, the virus was propagated for 48 h in the presence of 6 or 10 and virus titres were determined. At this inhibitor concentration, a reduction of 14 and 94% in virus titre by 6 and 10, respectively, was calculated ( Supplementary Fig. 6b ). Virus growth inhibition IC 50 values were then determined for the two inhibitors in a well-established in situ enzyme-linked immunosorbent assay (ELISA) technique [11] using three different cell lines. We chose LLC-MK2 (monkey kidney epithelial cells) cell line as it is extensively used in hPIV-3 cell-based infection studies [1] as well as the hPIV-3 susceptible human respiratory cell lines A549 (lung adenocarcinoma epithelial cells) [36] and normal human bronchial epithelial primary cells to investigate virus growth inhibition in natural tissue-related cells. The method itself has useful advantages over the virus titration method as it is a faster, one-step, non-subjective technique that correlates non-immobilized virus growth to HN expression levels of a low multiplicity of infection-infected cell monolayer. Interestingly, slightly lower virus growth inhibition IC 50 values were determined for 10 and 6 with the laboratory-established cell line LLC-MK2 in relation to the human cell lines. Overall, the same trend is observed for all the three cell lines in that a significantly stronger antiviral effect of inhibitor 10 (IC 50 =2.1–13.9 μM) is determined compared with inhibitor 6 (IC 50 =54.6–130.6 μM) ( Fig. 5 ). 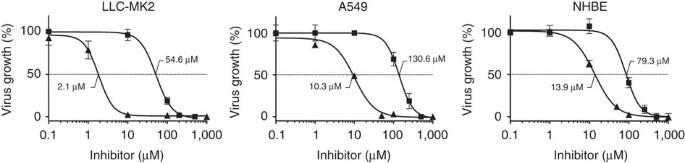Figure 5: Virus growth inhibition of the reference inhibitor 6 (▪) and inhibitor 10 (▴) in various cell lines. Virus growth IC50values of compounds6(▪) and10(▴) were determined by anin situELISA technique against both human cell lines (A549 and NHBE) and a monkey kidney cell line (LLC-MK2). IC50values of 54.6±3.8 μM and 2.1±0.6 μM (LLC-MK2); 130.6±13.0 μM and 10.3±0.3 μM (A549); 79.3±1.0 μM and 13.9±0.7 μM (NHBE) were determined for6and10,respectively. These values were determined from at least two independent experiments performed in triplicate and error bars correspond to the calculated s.d. Figure 5: Virus growth inhibition of the reference inhibitor 6 (▪) and inhibitor 10 ( ▴ ) in various cell lines. Virus growth IC 50 values of compounds 6 ( ▪ ) and 10 ( ▴ ) were determined by an in situ ELISA technique against both human cell lines (A549 and NHBE) and a monkey kidney cell line (LLC-MK2). IC 50 values of 54.6±3.8 μM and 2.1±0.6 μM (LLC-MK2); 130.6±13.0 μM and 10.3±0.3 μM (A549); 79.3±1.0 μM and 13.9±0.7 μM (NHBE) were determined for 6 and 10, respectively. These values were determined from at least two independent experiments performed in triplicate and error bars correspond to the calculated s.d. Full size image Structural biology Saturation Transfer Difference (STD) NMR experiments of 8 in complex with recombinantly expressed hPIV-3 HN ( Supplementary Fig. 7 ) and the most potent inhibitor 10 in complex with either recombinantly expressed hPIV-3 HN ( Fig. 6 ) or intact hPIV-3 virus ( Supplementary Fig. 8 ) were undertaken to further support our computational and biological studies that demonstrated specific binding and inhibition. 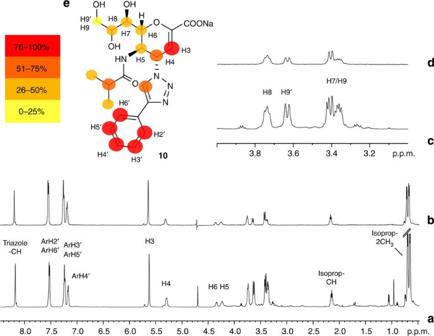Figure 6:1H and STD NMR spectra and epitope map of10in complex with hPIV-3 HN. (a)1H NMR spectrum of10. (b) STD NMR spectrum of10in the presence of 20 μM hPIV-3 HN at a protein:ligand ratio of 1:100 (2 mM of10). (c)1H NMR spectrum of the H7, H8, H9 and H9′ regions. (d) STD NMR spectrum of the H7, H8, H9 and H9′ regions. (e) Proposed binding epitope map of inhibitor10. Figure 6: 1 H and STD NMR spectra and epitope map of 10 in complex with hPIV-3 HN. ( a ) 1 H NMR spectrum of 10 . ( b ) STD NMR spectrum of 10 in the presence of 20 μM hPIV-3 HN at a protein:ligand ratio of 1:100 (2 mM of 10 ). ( c ) 1 H NMR spectrum of the H7, H8, H9 and H9′ regions. ( d ) STD NMR spectrum of the H7, H8, H9 and H9′ regions. ( e ) Proposed binding epitope map of inhibitor 10 . Full size image STD NMR signal intensities for all protons associated with 8 or 10 were clearly observed, to varying extents, when the inhibitor is in complex with either intact virus or recombinant hPIV-3 HN and clearly demonstrated that the ligand binds in both instances. The minor signals visible at 3.25, 3.5 and 4.0 p.p.m. in the 1 H NMR spectrum of 10 acquired in the presence of intact virus particles were a consequence of impurities from the virus purification process and belong to neither the virus particles nor 10 . As anticipated, none of these signals were observed in the STD NMR spectrum and clearly demonstrate that the impurities do not bind to the virus ( Supplementary Fig. 8 ). These experiments clearly demonstrate the specific binding of 10 to both intact hPIV-3 virus and hPIV-3 HN, further substantiating the inhibitor’s biological relevance and potential. Importantly, an overlay of the aromatic phenyl protons signals observed at 7.1–7.6 p.p.m. in the STD NMR spectra for both the intact virus and recombinant HN protein also reveals that the binding epitope of inhibitor 10 is similar, if not identical, when bound either to intact hPIV-3 virus or to recombinant hPIV-3 HN protein ( Supplementary Fig. 9 ). Epitope mapping of inhibitor 10 A complete ligand-binding epitope was determined by the analysis of STD NMR spectra ( Fig. 6 ) of hPIV-3 HN protein in complex with 10 . All STD NMR signals of 10 were normalized to the strongest STD NMR signal observed, the inhibitor’s H4′ proton at 7.18 p.p.m. Relative STD NMR effects for all protons of the inhibitor were then calculated ( Supplementary Table 3 ). The extent of the STD NMR signal intensity strongly depends on the proton’s proximity to the protein surface and reveals how the designed inhibitor 10 engages the HN protein’s binding site. Notably, very strong relative STD NMR effects were observed for the phenyl group protons H2′, H3′, H4′, H5′and H6′ between 7.1 and 7.6 p.p.m. revealing a close contact in that region of the molecule to the protein surface. Moreover, a significant STD NMR effect was likewise detected for the CH of the triazole moiety. In contrast, the C5 isobutyramido moiety’s protons of the inhibitor showed less effect (relative STD NMR signal intensities in the range of 42–54%). Interestingly, the protons associated with the Neu5Ac2en core structure of 10 displayed variable relative STD NMR effects. A significant H3-relative STD NMR signal intensity (80%) suggests a strong interaction of this part of the molecule with hPIV-3 HN. Furthermore, relative STD NMR signal intensities for H4, H5 and H6 of 59, 50 and 49%, respectively, demonstrate that the ring protons of the Neu5Ac2en core structure are also involved in inhibitor engagement to the protein. Finally, weaker relative STD NMR effects of 36, 35, 24 and 21%, were observed for the glycerol side chain protons H7, H8, H9 and H9′, respectively, and suggest that the glycerol side chain makes less of a contribution to the inhibitor-binding event compared with the C4 triazolo functionality and the inhibitor’s core ring structure ( Fig. 6 ). The inhibitor 8 epitope map ( Supplementary Fig. 7 ) was for all intents and purposes identical to that of inhibitor 10 , with the C4 triazolo moiety clearly in close contact to the protein surface. We have utilized MD simulations to verify the possibility, and to design and study the effect, of accommodating a Neu5Ac2en-based inhibitor with a bulky C4 substituent in the binding pocket of hPIV-3 HN. Previous MD studies [24] on this protein have demonstrated the existence of a flexible loop, the 216 loop, which can adopt an open conformation creating a larger cavity in the region of the Neu5Ac2en C4 hydroxyl group. Our detailed MD simulations in the current study clearly demonstrate that substantially larger substituents at the C4 position of Neu5Ac2en ( 2 ) may be accommodated in the hPIV-3 HN’s active site. The accommodation of bulkier C4 substituents is achieved by the C4 functionality occupying the 216 cavity and locking open the 216 loop. Furthermore, our simulations predict that the binding of such C4-functionalized inhibitors is highly efficient and should result in potent inhibition of hPIV-3 HN. For example, a Δ E avI of −212.50 kJ mol −1 between 10 and the extensively studied neuraminidase inhibitor 2 in complex with hPIV-3 HN was calculated and confirms the positive influence on E avI for the combined C4/C5 modification on the Neu5Ac2en template. To experimentally validate our theoretical predictions, we successfully synthesized, in less than 10 steps, the designed C4- and C5-functionalized Neu5Ac2en inhibitors 8 and 10 from commercially available starting materials in very good overall yield. Our synthetic strategy towards these novel inhibitors provides great versatility for additional functionalization and enables further exploration of the Neu5Ac2en template in inhibitor optimization studies. The biological evaluation of the reference and novel designer C4- and C5-functionalized Neu5Ac2en inhibitors using protein-based inhibition assays (NI and HI) led to a number of conclusions concerning the influence of C4 and C5 substituents on inhibitor potency. Within each of the two screened groups, that is Group 1 (C5 acetamido) and Group 2 (C5 isobutyramido), the order of potency based on the substituent at C4 was found to be as follows: hydroxyl<azido≤4-methoxymethyltriazole<4-phenyltriazole. The weakest inhibition in both groups was observed for the 4-hydroxy derivatives 2 and 5 . This outcome supports the notion that the C4-binding domain, which accommodates the C4 hydroxyl group on Neu5Ac2en ( 2 ), has significant hydrophobic character and consequently does not favour the interaction with a polar, hydrophilic group including a hydroxyl group [25] . The hydrophobic nature of the pocket, combined with the large 216 cavity size created by the opening of the 216 loop, does favour inhibitors, including inhibitors 8 and 10 , which have the C4 hydroxyl group replaced with bulky hydrophobic substituents. Comparison of both group’s IC 50 values ( Fig. 4 ) revealed that replacement of the C5 acetamido group with an isobutyramido group in all of the prepared inhibitors led to overall enhanced potency. Typically, close to an order of magnitude improvement was observed, except for the most potent inhibitor 10 . Furthermore, analysis of the IC 50 values ( Fig. 4 ) supports the notion that the potency enhancement in the best inhibitors, 8 and 10 , results predominantly from the introduction of the C4 substituent, with the C5 substituent contributing to a much lesser extent. This notion is also substantiated by STD NMR data analysis ( Fig. 6 ) that led to an epitope map of inhibitor 10 in which the protons of the 4-phenyltriazole moiety showed the strongest contribution to the binding event of 10 in complex with hPIV-3 HN, while the relative interactions observed for the isobutyramido group were significantly less ( ∼ 50%). Further comparison of the various groups of inhibitors provided relative IC 50 improvement factors for both NI and HI as detailed ( Supplementary Fig. 4 ). Interestingly, a comparison of the parent templates 2 and 5 , which contain a C4 hydroxyl group, with their corresponding C4-functionalized derivatives 8 and 10, respectively, shows dramatic HI improvement on C4 functionalization. The trend in the increase in NI is similar to that observed for HI; for example, inhibitors 5 , 6 and 9 had a 5–20-fold enhancement in potency by increasing the size of the C5 substituent from an acetamido to an isobutyramido functionality. However, a comparison of the potential NI and HI improvement factors also suggests that when a bulky C4 substituent is present, as in 8 and 10 , the introduction of the bulkier C5 isobutyramido moiety ( 10 ) improves potency to a lesser extent, by only a factor of two to three compared with the acetamido moiety ( 8 ). The consequence of locking the 216 cavity open by the bulky C4-functionalized derivative is positional changes of amino acid side chains associated with the active site domains that recognize the C4 and C5 functionalities on N -acetylneuraminic acid ( 1 ) and its various unsaturated derivatives. These changes appear to equally accommodate the smaller C5 acetamido substituent and the bulkier C5 isobutyramido functionality. The potent inhibition of both HN functions (NI and HI) by inhibitor 10 demonstrates that the compound exerts its antiviral effect against hPIV-3 by action on the virus’ key HN protein. These findings are further supported by STD NMR experiments of 10 in complex with either the intact virus or the recombinant HN protein, which clearly show identical STD NMR signal intensities for the inhibitor’s C4 triazole aromatic moiety ( Supplementary Figs 8 and 9 ). Moreover, the calculated binding epitope for 10 in complex with hPIV-3 HN ( Supplementary Table 3 ) is in excellent agreement with our MD simulations that clearly predict the close contact of the Neu5Ac2en derivative’s H3 and the C4 triazolo moiety’s phenyl protons to the protein surface ( Fig. 3c ). Furthermore, the in situ ELISA results ( Fig. 5 ) were in good agreement with the NI and HI assay data. Interestingly, the LLC-MK2 cell-based assays demonstrated that 10 is even more potent at the cellular level compared with NI and HI protein-based assays. In this cell-based assay, 10 was found to be ∼ 26 times more potent than 6 , whereas protein inhibition assays showed only ∼ 8 and 11-fold improvement in NI and HI assays, respectively ( Supplementary Fig. 4 ). This strongly suggests that 10 is a potent dual-acting inhibitor that derives efficient synergism from the inhibition of both the protein’s neuraminidase and haemagglutinin activities. This is in contrast to the previously reported inhibitor 6 , which derives less synergistic effect as a result of its significantly poorer inhibition of the haemagglutinin activity. Finally, the extent of virus growth inhibition in both human cell lines for inhibitor 10 compared with 6 clearly demonstrates the superiority of the designer ligand 10 ( Fig. 5 ). In conclusion, we have taken advantage of the hPIV-3 HN 216 loop flexibility [24] . On the basis of the notion that the 216 cavity, created by loop movement, is of sufficient size to accommodate larger functionalities at C4 on the Neu5Ac2en-based template, we designed and synthesized inhibitors 7 – 10 that incorporate a bulky substituted triazolo substituent at C4. Our predicted efficient occupation of the HN active site and the proposed 216 cavity by these new bulky inhibitors translated to potent inhibition of both HN functions, as well as significant blockade of virus propagation. Moreover, our predicted trend in overall interaction energies of inhibitors 2 , 8 and 10 with hPIV-3 HN is confirmed by experimentally determined IC 50 values and further demonstrates the power of structure-guided inhibitor design. The novel designer potent inhibitor 10 efficiently locks open the 216 loop and provides an exciting template for further hPIV-3 HN dual-acting inhibitor development. Finally, we have found that these inhibitors efficiently block both virus cell entry and virion progeny release and provide new direction towards anti-parainfluenza drug development. MD simulations MD simulations were performed with GROMOS software [37] , [38] using the force-field parameter set 54A4 (ref. 39 ). Initial coordinates were taken from the X-ray structure (PDB accession code 1V3E ) (ref. 25 ) of hPIV-3 HN in complex with 4 . Compound 8 has been superimposed on zanamivir ( 4 ) ring atoms from the crystal structure. Parameters for 8 were generated in an analogous manner [40] to existing parameters in the GROMOS force field ( Supplementary Table 1a–e ). The number of atoms in the final composite system for 1V3E– 4 and IV3E– 8 was 78,253 and 78,084, respectively. Ionization states of amino acid residues were assigned at pH 7.0. The histidine side chains were protonated at the N ɛ atom. Water molecules associated with the X-ray structure were removed, and replaced by explicit solvation using the simple point charge water model [41] and periodic boundary conditions, consistent with our previously published methodology [24] . In the simulations, water molecules were added around the protein within a truncated octahedron with a minimum distance of 1.4 nm between the protein atoms and the square walls of the periodic box. All bonds were constrained with a geometric tolerance of 10 −4 using the SHAKE algorithm [42] . A steepest descent energy minimization of the system was performed to relax the solute–solvent contacts while positionally restraining the solute atoms using a harmonic interaction with a force constant of 2.5 × 10 4 kJ mol −1 nm −2 . Next, steepest descent energy minimization of the system without any restraints was performed to eliminate any residual strain. The energy minimizations were terminated when the energy change per step became smaller than 0.1 kJ mol −1 . For non-bonded interactions, a triple-range method with cutoff radii of 0.8/1.4 nm was used. Short-range van der Waals and electrostatic interactions were evaluated at each time step, based on a charge-group pair list. Medium-range van der Waals and electrostatic interactions, between (charge group) pairs at a distance longer than 0.8 nm and shorter than 1.4 nm, were evaluated every fifth time step, at which point the pair list was updated. Outside the longer cutoff radius, a reaction-field approximation [43] was used with a relative dielectric permittivity of 78.5. The centre of mass motion of the whole system was removed every 1,000 time steps. Solvent and solute were independently weakly coupled to a temperature bath of 295 K with a relaxation time of 0.1 ps (ref. 44 ). The systems were also weakly coupled to a pressure bath of 1 atm with a relaxation time of 0.5 ps and an isothermal compressibility of 0.7513 × 10 −3 (kJ mol −1 nm −3 ) −1 . MD simulations of 20 ps periods with harmonic position restraining of the solute atoms and force constants of 2.5 × 10 4 , 2.5 × 10 3 , 2.5 × 10 2 and 2.5 × 10 1 kJ mol −1 nm −2 were performed to further equilibrate the systems at 50, 120, 180, 240 and 300 K, respectively. The simulations were each carried out for 30 ns. The trajectory coordinates and energies were saved every 0.5 ps for analysis. Simulation trajectories for hPIV-3 HN in complex with 4 were produced in an analogous manner to that described above [24] and were used for analysis and comparison of results obtained for hPIV-3 HN in complex with 8 . Analyses were done with the analysis software GROMOS++ (ref. 45 ). Atom-positional r.m.s.d. between structures were calculated for the residues comprising the 216 loop (residues 210–221) by performing a rotational and translational atom-positional least-squares fit of one structure on the second (reference) structure using a given set of atoms (N, C α , C). Atom-positional r.m.s.f. were calculated as an average from a 30-ns period of simulation by performing a rotational and translational atom-positional least-squares fit of the C α atoms of the trajectory structures on the reference. r.m.s.f. were calculated for all residues including the 216 loop (residues 210–221). To obtain reduced, representative structural ensembles for the simulations, r.m.s.d.-based conformational clustering was performed [46] . Structures extracted every 10 ps from simulations were superimposed on backbone-C α atoms to remove overall rotation and translation. Clustering of all atoms of residues that line the binding site (residues 190–198, 210–221, 251–259, 274–280, 320–326, 334–339, 369–377, 407–413, 474–480 and 529–533) was performed to compare relative structural populations of hPIV-3 HN protein from the different simulation trajectories. The similarity criterion applied was the r.m.s.d. of all atoms of these residues with a cutoff of 0.13 nm. Final structures resulting from the 30 ns of MD simulations were extracted. Interaction energies between hPIV-3 HN and inhibitors 8 and 10 were calculated using GROMOS generated energies, free-energy λ derivatives and block averages as separate trajectory files, referred to as the energy trajectory [45] . The programme ene_ana [45] was used to extract individual interaction energy values such as non-bonded contributions, that is, van der Waals and Coulomb interactions from these files. Thus, these contributions between the ligand and the protein were extracted from the energy trajectory resulting from the simulation and interaction energies calculated. The error estimate was calculated from block averages of growing sizes extrapolating to infinite block size. Hydrophobic interactions were analysed and a map of interactions between inhibitor 10 and hPIV-3 HN was created using LIGPLOT [47] . To measure the extent of cavity opening for selected structures, the pocket volume was analysed using POVME [48] . Importantly, extended simulation times, up to 80 ns provided outcomes entirely consistent with the data presented. Chemistry Synthesis of intermediates . The synthesis of intermediates 11 (ref. 28 ), 12 (ref. 29 ) and 17 – 24 (ref. 29 ) and reference inhibitors 2 (ref. 49 ), 3 (ref. 50 ), 5 (ref. 29 ) and 6 (ref. 29 ) was achieved by the relevant literature procedure. General methods are described in the Supplementary Methods . General procedure for the synthesis of 18 and 19 . A mixture of 17 or 11 (0.42 mmol), Boc 2 O (275 mg, 1.27 mmol) and 4-Dimethylaminopyridine (50 mg, 0.42 mmol) in anhydrous tetrahydrofuran (5 ml) was stirred under argon atmosphere at 60 °C o/n ( Supplementary Fig. 1 ). After cooling to RT, the solvent was evaporated under vacuum, and the residue was taken up in dichloromethane (DCM) for chromatographic separation on a silica gel column using ethyl acetate:hexane (1:2) as solvent to yield pure 18 (170 mg, 71%) or 19 (225 mg, 96%). General procedure for the synthesis of 20 and 21 . To a methanolic solution of NaOMe, freshly prepared by dissolving sodium metal (0.39 mmol, 9 mg) in anhydrous MeOH (5 ml), was added compound 18 or 19 (0.26 mmol) ( Supplementary Fig. 1 ). The mixture was stirred at RT for 1 h and then quenched with Amberlite IR-120 (H + ) resin (to pH=5). The resin was filtered off, washed with MeOH (5 ml × 3) and the combined filtrate and washings were evaporated under vacuum. The residue was redissolved in pyridine (2 ml), and acetic anhydride (0.5 ml) added. The reaction mixture was stirred at RT under argon atmosphere o/n and the solvent and excess Ac 2 O were then removed under vacuum. Finally, the residue was taken up in DCM for chromatographic separation on a silica gel column using ethyl acetate:hexane (1:2) as solvent to yield pure 20 (112 mg, 81%) or 21 (84 mg, 63%). General procedure for the synthesis of 22 and 23 . To a solution of 20 or 21 (0.15 mmol) in anhydrous DCM (2 ml) was added TFA (230 μl, 3.0 mmol) and the mixture was stirred at RT under argon o/n ( Supplementary Fig. 1 ). The reaction was diluted with DCM (20 ml) and quenched with saturated aqueous NaHCO 3 solution (20 ml). The DCM layer was washed with water and brine and then dried over anhydrous Na 2 SO 4 . The dried organic solvent was concentrated under vacuum, and purified by silica gel chromatography using the suitable solvent system to yield pure 22 (58 mg, 90%) or 23 (53 mg, 85%). General procedure for the synthesis of 24 and 12 . To a solution of 22 or 23 (0.116 mmol) in DCM (2 ml) under argon was added Et 3 N (82 μl, 0.58 mmol) and isobutyryl chloride (18 μl, 0.17 mmol; Supplementary Fig. 1 ). The mixture was stirred at RT for 4 h and then loaded on a silica gel column for chromatographic separation using ethyl acetate:hexane (1:1) as solvent to yield pure 24 (50 mg, 84%) or 12 (51 mg, 91%). General procedure for the synthesis of 5 and 6 . To a suspension of compound 24 or 12 (0.08 mmol) in a 1:1 mixture of MeOH:H 2 O (2 ml) at 0 °C was added dropwise a NaOH solution (1.0 M) until pH ∼ 14 ( Supplementary Fig. 1 ). The temperature was raised gradually to RT and the mixture was stirred at RT overnight. The solution was then acidified with Amberlite IR-120 (H + ) resin (to pH=5), filtered and washed with MeOH (10 ml) and H 2 O (10 ml). The combined filtrate and washings were then concentrated under vacuum and the residue was diluted with distilled water (5 ml) and adjusted to pH=8.0 using 0.05 M NaOH to convert the compound to its sodium salt. The compounds were then purified on a C18-GracePure cartridge using 2% acetonitrile/water as solvent to yield pure 5 (26 mg, 94%) or 6 (24 mg, 82%) as fluffy white powders. General procedure for the synthesis of 13 – 16 . The appropriate 4-azido-4-deoxy-Neu5Ac2en derivative ( 11 or 12 , 0.22 mmol) and the corresponding ethynyl derivative (0.33 mmol) were dissolved in a 1:1 mixture of tert -butanol:H 2 O (4 ml; Supplementary Fig. 2 ). Copper(II) sulfate pentahydrate (4 mg, 0.015 mmol) was added to the mixture followed by sodium ascorbate (0.1 ml of freshly prepared 1 M solution in H 2 O). The mixture was stirred at 45 °C for 6 h and then left to cool at RT. The mixture was then diluted with DCM (100 ml), washed with 10% NH 4 OH (50 ml), followed by brine (50 ml). The organic layer was dried over anhydrous Na 2 SO 4 and concentrated under vacuum to give the crude products 13 – 16 , which were purified by silica gel chromatography using an appropriate solvent system ( Supplementary Methods ). General procedure for the synthesis of 7 – 10 . To a suspension of the protected triazole derivative 13 – 16 in a 1:1 mixture of MeOH:H 2 O (2 ml) at 0 °C was added dropwise a NaOH solution (1.0 M) until pH ∼ 14 ( Supplementary Fig. 2 ). The temperature was gradually raised to RT and the mixture was stirred at RT overnight. The solution was then acidified with Amberlite IR-120 (H + ) resin (to pH=5), filtered and washed with MeOH (10 ml) and H 2 O (10 ml). The combined filtrate and washings were then concentrated under vacuum, then diluted with distilled water (5 ml) and adjusted to pH=8.0 using 0.05 M NaOH to convert the compound to its sodium salt. Finally, the compound was purified on a C18-GracePure cartridge using 2% acetonitrile/water as solvent to yield the pure products 7 – 10 . All novel compounds were appropriately characterized and were of high purity ( Supplementary Methods and Supplementary Fig. 3a–t ). Biology Cells and virus . A549 cells (adenocarcinomic human alveolar basal epithelial cells) were provided by the European Collection of Cell Cultures (86012804-1VL, Sigma-Aldrich). Cells were propagated in Dulbecco's Modified Eagle Medium (Lonza, Basel, Switzerland) supplemented with 1% Glutamine (200 mM) and 5% fetal bovine serum. For infection and post-infection procedures, A549 cells were maintained in Dulbecco's Modified Eagle Medium supplemented with 1% Glutamine only. Normal human bronchial/tracheal epithelial cells (CC-2540, lot 313831, Lonza) were amplified in B-ALI growth medium (Lonza) and the same medium was used for infection and post-infection studies. LLC-MK2 cells (Rhesus monkey kidney, ATCC CCL-7) were cultured in Eagle's minimal essential medium (EMEM) (Lonza) supplemented with 1% Glutamine (200 mM) and 2% of heat-inactivated fetal bovine serum. During hPIV-3 infection and post-infection incubation, LLC-MK2 cells were maintained in EMEM supplemented with 1% glutamine. All cell lines were incubated at 37 °C in a humidified atmosphere of 5% CO 2 . hPIV-3 (strain C-243) was obtained from the American Type Culture Collection (ATCC, Manassas, VA). The virus was propagated in LLC-MK2 cells with EMEM supplemented with glutamine (EMEM inf ) at 35 °C in a humidified atmosphere of 5% CO 2 . Virus-containing culture supernatant was collected 3 to 4 days post infection, while monitoring cytopathic effects, and clarified from cell debris by centrifugation (3,000 r.c.f. for 15 min). Virus was concentrated at least 10 times using 30 kDa Amicon Ultra filter unit (Millipore, Billerica, MA) for use in HI assays. NI assays and STD NMR experiments used virus that was polyethylene glycol (PEG)-precipitated and then purified as described below. Clarified hPIV-3 supernatant was mixed with PEG6000 (8% final concentration) and NaCl (0.4 M final concentration) and then incubated overnight at 4 °C under gentle agitation. PEG6000/hPIV-3 complex was pelleted by centrifugation at 3,000 r.c.f. for 30 min at 4 °C. The supernatant was discarded and a volume of GNTE buffer (glycine, 200 mM, NaCl, 200 mM, Tris-HCl, 20 mM, EDTA, 2 mM, pH 7.4) corresponding to at least 1:40 of the initial virus suspension volume was used to resuspend the pellet overnight at 4 °C. The virus suspension was homogenized by up and down pipetting followed by a mechanical disruption of the remaining virus aggregates using a douncer with ‘tight' pestle. The hPIV-3 homogenate was loaded on top of a 30–60% non-linear sucrose gradient prepared in GNTE buffer and centrifuged at 100,000 r.c.f. for 2 h 30 min at 4 °C without brake for deceleration. The virus was concentrated at the 30–60% sucrose interface and then collected and stored at −80 °C for NI assays or at 4 °C for STD NMR experiments. Recombinant HN expression and purification . The peptide sequence of hPIV-3 prototype strain C-243 was used as a reference to design a secreted and soluble recombinant HN protein based on a substantially modified ( Supplementary Methods ) literature procedure [25] . HI assay . Both human (h RBC) and guinea pig red blood cells (gp RBC) were used in the HI assay [18] , [33] and had high agglutination efficiency ( Supplementary Methods ). NI assay . The purified hPIV-3 NA was assayed using a method adapted [50] ( Supplementary Methods ) from Potier et al . [30] and measured the relative fluorescence of 4-methylumbelliferone, the product of the enzymatic hydrolysis of MUN (Sigma-Aldrich, St Louis, MO). Virus growth inhibition assay . Before assessing the best inhibitors in cell-based assays, an MTT (3-(4,5-dimethylthiazol-2-yl)-2,5-diphenyltetrazolium bromide) assay was performed to evaluate the compound cytotoxicity. No cytotoxic effect was observed after incubation for 48 h of LLC-MK2 cells with 6 , 8 and 10 at 303 μM, the highest concentration tested. Virus growth inhibition was assessed using a focus-forming assay [51] by titration of progeny in the presence of 2 μM of 6 , 8 and 10 in EMEM inf from a low multiplicity of infection-infected confluent LLC-MK2 monolayer in a 48-well plate format. Virus inoculum (100 focus-forming units per well) was preincubated with 6 , 8 and 10 for 20 min. Infection was performed in duplicate and continued for 1 h at 37 °C with gentle agitation every 15 min. Inocula were removed and replaced with 500 μl per well of each respective 2 μM compound dilution (in EMEM inf ). A positive control for infection was included using the same conditions minus the compound. Virus proliferation on infected cell monolayers were maintained for 48 h at 37 °C, 5% CO 2 . Culture supernatants from duplicates were collected, pooled and clarified at 15,000 r.c.f. for 10 min and stored at −80 °C. Supernatants were diluted in EMEM inf by 10 −3 , 10 −4 and 10 −5 to avoid any remaining compound effect on the subsequent virus titration. Virus titrations were done in duplicate using the previously described conditions for virus infection. After 1 h, Avicel (FMC BioPolymer, Philadelphia, PA) in EMEM inf was directly added to the inoculum (1% final concentration) to restrict and localize virus proliferation. The plate was incubated for 36 to 40 h at 37 °C, 5% CO 2 to allow focus formation. Avicel was gently removed and replaced with 3.7% paraformaldehyde/PBS and the plate was then kept for 15 min at RT for virus inactivation and cell fixation. Cell monolayers were washed three times for 5 min each with PBS and then endogenous peroxidase inactivated with 0.3% H 2 O 2 /PBS for 30 min at 37 °C. The plate was washed again three times for 5 min each with PBS and incubated with mouse monoclonal IgG anti-hPIV-3 HN (Fitzgerald, clone# M02122321, 2.0 mg ml −1 ) at 1 μg ml −1 in 5% milk/PBS for 1 h at 37 °C. Cell monolayers were washed three times for 5 min with 0.02% Tween20/PBS. Goat anti-Mouse-IgG(H+L)-HRP conjugate (BioRad, ref# 170–6516) diluted at 1:1,000 in 5% milk/PBS was added to each well and incubated for 1 h at 37 °C. Cell monolayers were washed as previously described with 0.02% Tween20/PBS and then rinsed twice with PBS. Foci were revealed by adding TrueBlue solution (HRP substrate) on each well and incubating the plate for 1 h at 37 °C. The TrueBlue solution was discarded and the plate rinsed twice with water then dried before being scanned ( Supplementary Fig. 5 ) and foci counted. The IC 50 value was considered as the concentration of inhibitor that reduced the progeny virus titre by 50% compared with a non-treated infected LLC-MK2 monolayer. In situ ELISA . In situ ELISA is another technique used in drug discovery to evaluate virus growth inhibition [11] , [52] , [53] , [54] , [55] . This technique is highly sensitive and reliable as it measures, in one step, the expression level of hPIV-3 HN at the cell surface of an infected cell monolayer. The expression level is directly correlated to the ability of a non-immobilized virus to infect and reinfect target cells. Infection was performed on a confluent cell monolayer seeded in a 96-well plate. Virus (40 focus-forming units per well) was preincubated for 20 min with compound 6 and 10 at a final concentration from 1,000 μM to 0.001 μM as a 10-fold dilution series. Infection was done in triplicate and continued for 1 h at 37 °C with gentle agitation every 15 min. Inocula were removed and replaced with 200 μl per well of each respective compound dilution. A positive control for infection was incorporated by the use of identical experimental conditions, minus inhibitor. Infected cell monolayers were kept for 36–40 h at 37 °C, 5% CO 2 for virus proliferation. Virus was inactivated and cells fixed by the direct addition of 100 μl of 11.1% paraformaldehyde/PBS. The plate was maintained at RT for 15 min and then washed 3 times for 5 min with PBS and then endogenous peroxidases were inactivated by treatment with 0.3% H 2 O 2 /PBS for 30 min at 37 °C. The cell monolayers were washed and incubated with mouse monoclonal IgG anti-hPIV-3 HN (Fitzgerald, clone# M02122321, 2.0 mg ml −1 ) at 1 μg ml −1 in 5% milk/PBS for 1 h at 37 °C. The wells were washed three times for 5 min with 0.02% Tween20/PBS. Goat anti-Mouse-IgG(H+L)-HRP conjugate (BioRad, ref# 170–6516), diluted at 1:2,000 in 5% milk/PBS, was added to each well and incubated for 1 h at 37 °C. Cell monolayers were washed with 0.02% Tween20/PBS and then rinsed twice with PBS. BD OptEIA TMB substrate (BD Biosciences, San Jose, CA, 100 μl) was added to each well and the plate was then incubated at 37 °C. The enzymatic reaction was stopped after 3–5 min by the addition of 50 μl of 0.6 M of H 2 SO 4 per well. Raw data were obtained by reading the absorbance (OD) of each well at 450 nm for 0.1 s with a Victor 3 multilabel reader (PerkinElmer, Waltham, MA). Final ODs were obtained by subtraction of the negative control (non-infected cells) OD from the initial OD reading and the data analysed with GraphPadPrism4 (GraphPad Software, Inc., La Jolla, CA) to calculate IC 50 values (non-linear regression (curve fit), Dose–response inhibition, four-parameter logistic). The IC 50 value was considered as the concentration of inhibitor that reduced the absorbance at 450 nm by 50%, compared with a non-treated infected cell monolayer. Standard deviation calculations . Standard deviations were calculated with GraphPadPrism4 (GraphPad Software, Inc., La Jolla, CA). Structural biology Sample preparation and 1 H NMR experiments . All NMR experiments were performed on a 600 MHz NMR spectrometer (Bruker) equipped with a 5-mm TXI probe with triple axis gradients. Intact virus suspension or recombinant hPIV-3 HN were buffer exchanged against 50 mM deuterated sodium acetate, 5 mM CaCl 2 in D 2 O at pD 4.6 by ultrafiltration using an Amicon Filter Unit (Millipore) with a cutoff value of 30 or 10 kDa, respectively. For each experiment, 20 μM hPIV-3 HN protein and a protein:ligand molar ratio of 1:100 in a final volume of 200 μl was used. 1 H NMR spectra were acquired with 32 scans at 283 K, a 2-s relaxation delay over a spectral width of 6,000 Hz. An initial STD NMR experiment was performed on a complex between compound 10 and intact hPIV-3 virus and all subsequent STD NMR experiments were performed on compounds in complex with recombinant hPIV-3 HN protein. STD NMR experiments . The protein was saturated on-resonance at −1.0 p.p.m. and off-resonance at 300 p.p.m. with a cascade of 60 selective Gaussian-shaped pulses of 50 ms duration, resulting in a total saturation time of 3 s and the relaxation delay was set to 4 s. Each STD NMR experiment was acquired either with a total of 1,056 scans (recombinant hPIV-3 HN) or 1,512 scans (intact virus) and a WATERGATE sequence was used to suppress the residual HDO signal. A Spin-lock filter with 5 kHz strength and duration of 10 ms was applied to suppress protein background. Control STD NMR experiments were performed with an identical experimental setup and the same ligand concentration but in the absence of protein. On- and off-resonance spectra were stored and processed separately, and the final STD NMR spectra were obtained by subtracting the on- from the off-resonance spectra. All STD effects were quantified using the equation A STD =(I 0 −I sat )/I 0 =I STD /I 0 . Therefore, signal intensities of the STD NMR spectrum ( I STD ) were compared with the corresponding signal intensities of a reference spectrum ( I 0 ). The strongest STD signal in the spectrum was assigned to a value of 100% and used as a reference to calculate relative STD effects accordingly [56] , [57] , [58] . How to cite this article: Guillon, P. et al . Structure-guided discovery of potent and dual-acting human parainfluenza virus haemagglutinin–neuraminidase inhibitors. Nat. Commun. 5:5268 doi: 10.1038/ncomms6268 (2014).